Improved heat dissipation in gallium nitride light-emitting diodes with embedded graphene oxide pattern The future of solid-state lighting relies on how the performance parameters will be improved further for developing high-brightness light-emitting diodes. Eventually, heat removal is becoming a crucial issue because the requirement of high brightness necessitates high-operating current densities that would trigger more joule heating. Here we demonstrate that the embedded graphene oxide in a gallium nitride light-emitting diode alleviates the self-heating issues by virtue of its heat-spreading ability and reducing the thermal boundary resistance. The fabrication process involves the generation of scalable graphene oxide microscale patterns on a sapphire substrate, followed by its thermal reduction and epitaxial lateral overgrowth of gallium nitride in a metal-organic chemical vapour deposition system under one-step process. The device with embedded graphene oxide outperforms its conventional counterpart by emitting bright light with relatively low-junction temperature and thermal resistance. This facile strategy may enable integration of large-scale graphene into practical devices for effective heat removal. Gallium nitride (GaN)-visible light-emitting diodes (LEDs) have witnessed rapid advancements because of the demand for efficient full-colour displays and general illumination in tandem with the rising awareness levels about energy conservation [1] , [2] , [3] . Especially, the white-light sources based on InGaN/GaN multiquantum-well blue LED chip with phosphor coatings and/or a combination of red-, green- and blue-emitting LED chips on a monolithic platform are the most promising solid-state lighting devices on the verge of replacing conventional incandescent and fluorescent lamps [4] , [5] , [6] . Despite significant progress in recent years [5] , [6] , larger chip area and higher driving current are the critical factors yet to be best optimized for achieving higher luminous efficiency. To unlock the full potential of the devices operating under high currents, it is imperative to find solutions for effective heat dissipation, because the devices, when operated at high driving currents, not only produce high luminance but also inevitably generate significant amounts of heat [3] , [7] . It has been reported that the optical power or luminous efficacy is degraded with the increasing junction temperature ( T j ) due to the thermal activation of non-radiative electron–hole recombination and/or electrostatic discharge [7] , [8] , [9] . Moreover, the number of defects responsible for non-radiative recombination also increases with T j [10] . Thus, it is obvious that the heat generation during high driving currents in LEDs could eventually obstruct the device reliability and durability. A number of studies have proposed the use of vertical geometry on high-thermal-conductivity substrates to overcome the thermal issues in high-efficiency GaN-based LEDs [3] , [11] , [12] . This approach has a significant advantage in terms of substrate heat dissipation [3] , which is a key for the realization of bright and durable LEDs. However, there also exist several long-standing drawbacks such as low device yield, difficulty in separating the epitaxial layers from the single-crystal substrate, complicated fabrication processes and so on [7] , [9] , [13] . Consequently, the search for the development of an effective heat dissipation means is intensifying to realize a robust solid-state lighting device with long life time. Graphene has attracted a tremendous amount of attention over the past few years because of its two dimensionality and unique physical properties [14] , [15] , which advance the graphene a promising next-generation material of widespread technological applications such as high-speed transistors [16] , flexible transparent heaters [17] , electrical interconnects [18] and transparent conducting electrodes in optoelectronic devices [19] , [20] , [21] , [22] . Despite graphene’s many other remarkable properties, the high intrinsic thermal conductivity, largely contributed by phonon component as a result of strong bonding of the light carbon atoms, has been focused to be a key advantage for applications in microelectronics and optoelectronic and photonic devices to alleviate the heat dissipation problems [23] , [24] , [25] . Initial experiments showed room-temperature thermal conductivity values as high as 600 and 5300 W mK −1 , respectively, for supported and suspended single-layer graphene [25] , [26] , values far higher than the thermal conductivity of Si (145 W mK −1 ) and copper (~400 W mK −1 ). A recent study on encased graphene [27] , however, revealed that the thermal conductivity can be well below that of suspended graphene, but it strongly depends on the layer numbers [24] . Recently, graphene-based composites functioning as thermal interface materials for heat management in integrated circuits have been demonstrated [24] , [28] . Moreover, a research group from the University of California-Riverside conducted an inspiring experiment that demonstrated graphene-based lateral heat spreaders for high-power GaN transistors [29] . Regardless of these notable advances in graphene research, the practical implementation of graphene as heat spreader in optoelectronic devices has yet to be realized. Furthermore, the integration of graphene into GaN-based devices remains challenging as direct epitaxial growth of nitride materials on graphene is impossible due to the lack of chemical reactivity [30] . Motivated by these considerations, we present the first experimental investigation of direct epitaxial growth of GaN-based blue LEDs on the reduced graphene oxide (rGO) pattern. Herein, patterned rGO acts as a buffer layer for the epitaxial lateral overgrowth of high-quality GaN and provides a better heat dissipation due to its high thermal conductivity. Recently, Yi et al. [30] , [31] demonstrated the growth of GaN thin films and LEDs on graphene with the use of high-density zinc oxide nanowalls as an intermediate layer. This strategy was developed aiming the fabrication of transferrable LEDs. It should be noted that our work completely differs from the above approach in following aspects. First, a combination of photolithography and spray-coating methods enables us to produce a low-cost, scalable and processable rGO pattern on sapphire substrate. This approach does not require additional graphene transfer process. Second, we have succeeded in growing high-quality GaN epilayers directly on the rGO pattern without using additional intermediate layer. The results show that the embedded rGO pattern not only acts as heat-spreading layer but also aids the growth of single-crystal high-quality GaN, which as a consequence leads to superior electrical and optical performance of the ensuing LED compared with the one grown on sapphire (referred to be as conventional LED). Using transient thermal measurements, the T j and thermal resistance ( R th ) are studied in detail and the results are discussed contemplating the thermal boundary resistance (TBR). Growth and characteristics of rGO The key processes involved in the GaN template growth on the rGO pattern are schematically illustrated in Fig. 1 . In brief, the formation of circular photoresist arrays and the deposition of graphene oxide dispersion on a sapphire substrate are accomplished using photolithography and the airbrush spray system [32] . Subsequent removal of photoresist results in the formation of hole patterns on the entire graphene oxide-covered substrate. Thereafter, an in situ thermal annealing process is carried out at 1100 °C under H 2 ambient for 10 min to reduce the graphene oxide, before the GaN is directly grown on this pattern in a metal-organic chemical vapour deposition reactor (see Methods for more details). Figure 2 shows the surface topography of graphene oxide-pattern-covered sapphire substrate before and after the thermal reduction process. 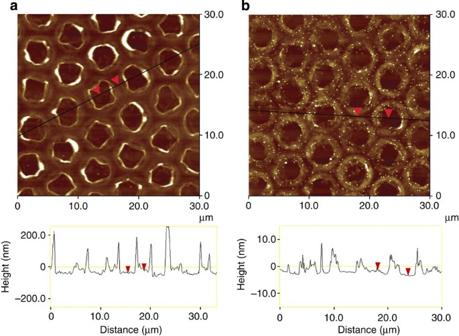Figure 2: AFM images of graphene oxide patterns produced on the sapphire. (a) Surface topography of graphene oxide patterns before thermal reduction process. The graphene oxide film is piled up (as high as 200 nm) around the circular hole pattern during the photoresist removal process. (b) Representative surface topography of a graphene oxide film subjected to annealing at 1100 °C for 10 min in a metal-organic chemical vapour deposition reactor. The height profiles obtained along the solid black lines marked in the images are provided under respective images. The red arrows in each image represent two selected points at which the vertical height difference gives a direct measure of the graphene oxide thickness. As can be seen from Fig. 2a , the spray method under optimized conditions gives highly adhered graphene oxide deposition over large area, and the photoresist removal process has no adverse effect on the deposits. The graphene oxide flakes are mainly arranged parallel to the substrate, and the thickness of the film was estimated to be approximately 15 nm. The morphology corresponding to the modified graphene oxide pattern after the thermal reduction is illustrated in Fig. 2b . One can notice a significant reduction in the film thickness (down to 2.2 nm) following the thermal reduction process ( Fig. 2b , sectional analysis). This is attributed to the shrinking of interlayer space because of the removal of the functional groups in the form of C-O and C=O [33] . It should be noted that the spray method is more appropriate for the photoresist-assisted graphene oxide pattern formation compared with the conventional spin coating, because the former involves deposition onto a heated substrate, which renders the deposit well adhered to the substrate. 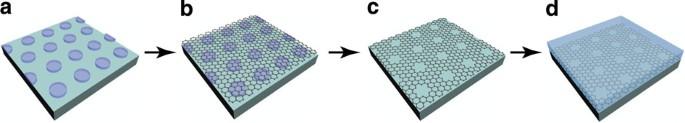Another advantage of this method is that it consumes only a small amount of solution even for large-scale deposition. Figure 1: Schematic of the key steps involved in the process of formation of graphene oxide-embedded LED. (a) The formation of circular arrays of photoresist masks on the sapphire substrate by photolithography process. (b) Deposition of graphene oxide on the sapphire substrate by the spray-coating method. (c) Removal of photoresist using acetone (during this step the graphene oxide film with arrays of hole patterns is created). (d) Thermal reduction and direct growth of GaN epilayer structure on the rGO pattern (here the hole arrays made on the graphene oxide facilitates the direct growth of GaN). Figure 1: Schematic of the key steps involved in the process of formation of graphene oxide-embedded LED. ( a ) The formation of circular arrays of photoresist masks on the sapphire substrate by photolithography process. ( b ) Deposition of graphene oxide on the sapphire substrate by the spray-coating method. ( c ) Removal of photoresist using acetone (during this step the graphene oxide film with arrays of hole patterns is created). ( d ) Thermal reduction and direct growth of GaN epilayer structure on the rGO pattern (here the hole arrays made on the graphene oxide facilitates the direct growth of GaN). Full size image Figure 2: AFM images of graphene oxide patterns produced on the sapphire. ( a ) Surface topography of graphene oxide patterns before thermal reduction process. The graphene oxide film is piled up (as high as 200 nm) around the circular hole pattern during the photoresist removal process. ( b ) Representative surface topography of a graphene oxide film subjected to annealing at 1100 °C for 10 min in a metal-organic chemical vapour deposition reactor. The height profiles obtained along the solid black lines marked in the images are provided under respective images. The red arrows in each image represent two selected points at which the vertical height difference gives a direct measure of the graphene oxide thickness. Full size image The C1s core-level spectra of X-ray photoelectron spectroscopy were used for the chemical analysis of the graphene oxide pattern before and after thermal reduction. Herein, curve fitting of the C1s spectra was performed using a Gaussian–Lorentzian peak shape after performing a Shirley background correction. The C1s spectrum ( Fig. 3a ) clearly indicates a considerable degree of oxidation with three components that correspond to carbon atoms in different functional groups: the C-C bond (284.5 eV) of sp 2 carbon in the basal plane of graphene oxide, the C in C-O bonds (286.6 eV), the carbonyls (C=O) bonds (288.2 eV) and carboxylates (O-C=O) bonds (289.2 eV) [34] . This can be further evidenced from the significant intensity levels of C-O and C=O peaks in the spectrum. After thermal reduction, the intensities of the respective peaks are significantly reduced ( Fig. 3b ), and the percentage of deoxidized carbon (C-C) is estimated to be 83%, which is much higher than the value (63%) estimated for the pristine graphene oxide. It is worthy to note that the former value is comparable to the values reported for chemically and thermally rGO [35] , [36] . 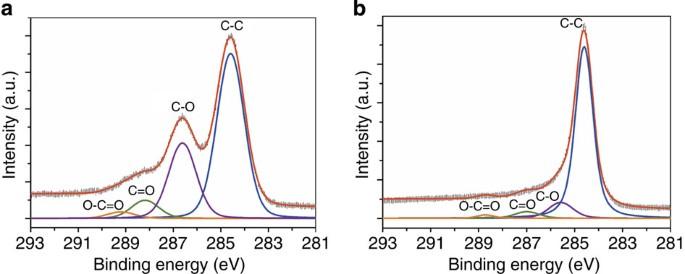Figure 3: C1s core-level spectra of graphene oxide pattern. (a) Before thermal reduction. (b) After thermal reduction. The different functional groups of carbon are shown by fitting each spectrum into the possible number of peaks. Figure 3: C1s core-level spectra of graphene oxide pattern. ( a ) Before thermal reduction. ( b ) After thermal reduction. The different functional groups of carbon are shown by fitting each spectrum into the possible number of peaks. Full size image Structural quality of the GaN epilayer We also made a systematic study to understand the crystal quality and microstructure of the GaN epilayers directly grown on the rGO pattern. Our approach for the successful realization of rGO-embedded GaN template was based on the epitaxial lateral overgrowth mechanism [37] , [38] . With the rGO pattern, the GaN growth begins selectively at the exposed sapphire regions (see Supplementary Fig. S1 ). When growth time increases, the GaN mounds also increases in size and coalescence occurs owing to the epitaxial lateral overgrowth. After a growth time of 90 min, a mirror-like GaN film is obtained. From X-ray rocking curve analyses, the half widths of (0002) and (10–12) peaks of the GaN templates grown on rGO (planar sapphire) are found to be 232 (248) and 402 (560) arcsec, respectively (see Supplementary Fig. S2 ). This signifies that the crystal quality of the GaN template grown on rGO pattern is comparatively better compared with the one grown on a sapphire substrate. Furthermore, the grown GaN template is found to be single crystalline, as shown in the cross-sectional high-resolution transmission electron microscopy (HR-TEM) images ( Fig. 4 ). The lattice spacing between the adjacent planes is measured to be 0.51 nm ( Fig. 4b ), corresponding to the d-spacing of (0001) plane of a wurtzite GaN crystal [39] . This result accompanied by the observed regular diffraction patterns further verified the single-crystalline nature of the GaN grown on the rGO pattern. The HR-TEM image also provides evidence that the rGO is embedded between the sapphire and GaN templates. From the average profile of intensity analysis ( Fig. 4d ), the thickness of the embedded rGO was estimated to be 2.5 nm, which is consistent with the atomic force microscopy (AFM) results. These results indicate the feasibility of using metal-organic chemical vapour deposition system for the effective reduction of graphene oxide and the simultaneous direct growth of GaN onto rGO in a single sequence. 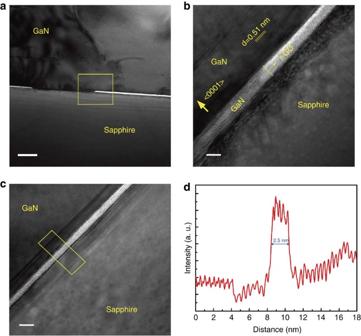Figure 4: TEM images of the rGO-embedded GaN template. (a) Cross-sectional bright field image of GaN/rGO/sapphire interface. Scale bar, 100 nm. (b,c) High-resolution snapshots of GaN/rGO/sapphire interface obtained in the rectangular region marked ina. The crystal plane direction and lattice spacing are marked in (b). Scale bar, 5 nm. (d) Average profile of intensity obtained in the rectangular region ofc. Figure 4: TEM images of the rGO-embedded GaN template. ( a ) Cross-sectional bright field image of GaN/rGO/sapphire interface. Scale bar, 100 nm. ( b , c ) High-resolution snapshots of GaN/rGO/sapphire interface obtained in the rectangular region marked in a . The crystal plane direction and lattice spacing are marked in ( b ). Scale bar, 5 nm. ( d ) Average profile of intensity obtained in the rectangular region of c . Full size image Infrared imaging of LED chip surface temperature This study has a particular spotlight on addressing the effective heat dissipation in graphene oxide-embedding LED chips. Hence, InGaN/GaN multiquantum-well blue LED chips with and without embedding the rGO pattern were fabricated (see Methods). First, the infrared imaging technique was used to monitor the temperature profile on the surface of the LED chips. To achieve a reliable data, the images were taken after waiting for a sufficiently long time to reach the thermal steady state. After processing the infrared camera images by (x, y) coordinates transformation, the infrared intensity images for the temperature distribution on the chip surface are obtained at 100 mA ( Fig. 5 ). The peak temperature of the chip surface rose up to 58 and 53.2 °C, respectively, for the conventional and rGO-embedded LEDs, measured within the same temperature range of 30–60 °C. In addition, the average temperature distribution on the chip surface is decreased for the rGO-embedded LED (47.06 °C) compared with its conventional counterpart (51.4 °C). This result signifies that with rGO at the GaN/sapphire interface, the heat generated in the interior of the chip is certainly reduced as compared with the conventional case. 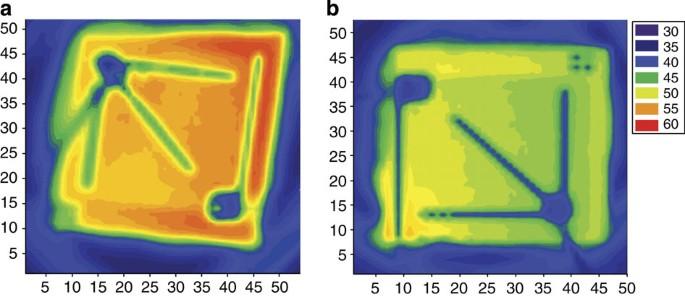Figure 5: Infrared thermal imaging camera photographs of the chip surfaces. (a) Temperature distribution on the surface of conventional LED chip. (b) Temperature distribution on the surface of rGO-embedded chip. The images are obtained under 100 mA current injections. The scale bar located at the right ofbgives an estimation of the temperature associated with different colours. Figure 5: Infrared thermal imaging camera photographs of the chip surfaces. ( a ) Temperature distribution on the surface of conventional LED chip. ( b ) Temperature distribution on the surface of rGO-embedded chip. The images are obtained under 100 mA current injections. The scale bar located at the right of b gives an estimation of the temperature associated with different colours. Full size image Transient thermal analysis of LED packages In LED packaging, T j and R th are the two physical quantities generally considered for the evaluation of heat dissipation. Therefore, to explore the extent of heat dissipation that the rGO can give, the above two parameters were studied using transient thermal analysis [40] , [41] (see Methods for more details). 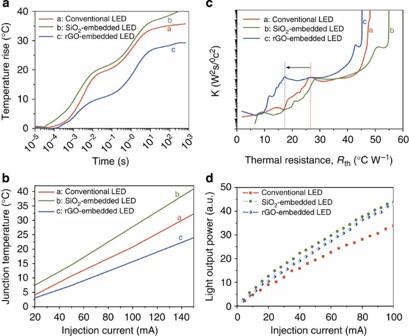Figure 6: Transient thermal and optical characteristics of different GaN LEDs. (a) Experimental transient cooling curves of the LED packages at an injection current of 150 mA. (b) Variations in junction temperature as a function of injection current. (c) Differential structure functions (K) of conventional, SiO2- and rGO-embedded LED packages under 150 mA current injections. (d) Light-output power of the LED chips as a function of injection current. Figure 6a shows the transient cooling curves of the LED packages obtained at 150 mA driving current. Here each curve represents time dependence of T j rise of a chip under a constant injection current. Figure 6b elucidates the measured T j as a function of injection current for the three LED packages under study. It should be noted that the T j increases with the injection current in all cases, a behaviour common to standard LED packages. For all the driving currents studied, the T j of the rGO-embedded LED is lower than its conventional counterpart. For instance, at 150 mA, the measured T j of the conventional and rGO-embedded LEDs are found to be 32.3 and 24 °C, respectively, indicating a 25.7% reduction in T j for the rGO-embedded LED. Figure 6: Transient thermal and optical characteristics of different GaN LEDs. ( a ) Experimental transient cooling curves of the LED packages at an injection current of 150 mA. ( b ) Variations in junction temperature as a function of injection current. ( c ) Differential structure functions (K) of conventional, SiO 2 - and rGO-embedded LED packages under 150 mA current injections. ( d ) Light-output power of the LED chips as a function of injection current. Full size image The differential structure functions that are derived by direct mathematical transformations from the experimental cooling curves are illustrated in Fig. 6c . Considering the chip as a sandwich structure, where the layers have the same area, the local peaks and valleys in the structure function denote reaching new materials in the heat-flow path. In Fig. 6c , the first peak denotes heat flow from chip to die-attach and the saturation region means heat flow from die-attach to heat-sink. In the structure functions shown in Fig. 6c , one can discriminate the characteristics of the two LED packages. Under a 150 mA current injection, the values of R th for the rGO-embedded and conventional LEDs are measured to be 17.3 and 26.2 °C W −1 , respectively. It is worthy to note that the R th of the rGO-embedded LED chip is lower by about 8.9 °C W −1 than its conventional counterpart. The reliability of the data was further verified by conducting measurements on a number of LED chips for each case under same experimental conditions. These results corroborate the infrared imaging observations and the T j results that the embedded rGO layer in the LED chip significantly improves the heat dissipation. Electrical and optical properties of GaN LEDs The electrical and optical characteristics of the rGO-embedded LED are compared with the conventional LED. The embedded rGO had no influence on the current-voltage characteristics of the device (see Supplementary Fig. S3 ). Figure 6d shows the variations in the light output power as a function of injection current. It is observed that the light output power of the rGO-embedded LED is slightly enhanced over that of conventional LED, which may be likely due to the improved internal quantum efficiency of the devices (see Supplementary Fig. S4 ). Additional experiments conducted to gain insights into the feasibility for high-power LEDs showed about 33% enhancement in the light output power at an injection current of 350 mA for the rGO-embedded LED (see Supplementary Fig. S5 ). Interestingly, the observed enhancement in the thermal and optical characteristics of the rGO-embedded LED is analogous to the results reported for vertical LEDs on graphite or Cu substrates [42] . Therefore, the present findings promise that graphene-based materials will soon find their way into high-power LEDs for thermal management. In general, heat generated in an LED flows along different paths primarily by conduction and convection processes. For conventional LED on sapphire, when the chip is mounted on a heat-sink, most of the heat flows from the active region through n-type cladding layer and the sapphire substrate to the heat-sink by conduction, and only a fraction of heat flows by convection means at surface-air boundaries [41] , [43] . In this structure, heat transfer to the heat-sink is slowed down because of the poor thermal conductivity of sapphire (38 W mK −1 ). This situation is different if there is a high-thermal-conductivity layer between the n-type cladding layer and sapphire substrate. Before addressing this later situation, it is necessary to clarify the issues associated with the thermal conductivity of graphene oxide. It is known that graphene oxide has different phonon dispersion and reduction never recovers graphene properties completely. The accurate thermal conductivity of the rGO is presently unknown. However, recent studies on the graphene-based thermal interface materials give strong evidences that chemically derived somewhat disordered graphene-multilayer graphene or graphene-few-layer graphene composites in flakes form could offer and preserve high thermal conductivity [28] , [44] . These benefits are known to originate from the disorder structure (in disordered materials, the thermal conductivity is found to increase with increasing temperature as a result of better phonon transmission through the interface and decreasing Kapitza resistance at high temperature) and the geometrical shape of the flake (well-ordered flakes of different sizes increase the thermal conductivity by the formation of better percolation network). Considering the above facts, it is reasonable to assume that a 2-nm thin rGO used in our experiments can have a considerable thermal conductivity, although it may not be as high as that of the few-layer graphene, which is known to exhibit thermal conductivity close to the bulk graphite limit of 2000 W mK −1 . Furthermore, the heat propagation along the in-plane direction of graphene being much larger than its perpendicular direction [23] , the embedded rGO is likely to ease out the heat from the chip by acting as a heat spreader. To understand the nature of the real mechanism by which heat dissipation occurs, a systematic study considering several other factors has been carried out. The GaN thickness is known to influence the heat spreading and associated temperature variations when GaN/substrate interface has large TBR [45] . However, the cross-sectional scanning electron microscopy images evidenced no major thickness difference between the samples grown simultaneously on planar sapphire and rGO buffer layer. The GaN epilayer quality can have a considerable impact on the lattice thermal conductivity that controls the heat flux on the GaN/substrate interface [46] , [47] . From the AFM analyses, the density values of the etch pits for the GaN epilayers grown on planar sapphire and rGO buffer layer are found to be 1.9 × 10 9 and 5.12 × 10 8 cm −2 , respectively. This result supports the HR X-ray diffraction measurements that the GaN crystal quality is significantly improved with the embedded rGO pattern, which certainly acted as a buffer layer to reduce the number of lattice defects that would propagate up to the critical GaN layers. Experimental and simulation studies emphasized that the dislocation density in a GaN layer must be at least of the order of the etch pits’ density [48] , [49] . The dislocation density being in the order of 10 8 –10 9 cm −2 , it is unrealistic to expect any significant variations in the thermal conductivity of the GaN, because the thermal conductivity is less sensitive to the dislocation density variations for values <10 11 cm −2 [46] . Therefore, an 8.9 °C W −1 reduction in the R th for the rGO-embedded LED cannot be attributed to only crystal quality enhancement. To comprehend the prime mechanism at play, a similar LED epilayer structure was grown on a low-thermal-conductivity amorphous SiO 2 buffer layer with patterns analogous to that of the rGO patterns used in our experiments. The benefit of this device design is that it can help to understand the impact of thermal conductivity of the buffer layer on the heat spreading. All the factors studied above were taken into consideration. Both the GaN thickness and the etch pit density (4.68 × 10 8 cm −2 ) are found to be comparable to that of the values observed for the sample grown with rGO buffer layer. However, a clue for the explication was from the transient thermal measurements, which indicated surprisingly very high R th (28.4 °C W −1 ) and T j (40.9 °C) for the device grown on SiO 2 buffer layer (see Fig. 6b and c ). If crystal quality improvement was the reason then devices grown on either of the buffer layers would have comparable T j and R th values. We surmise that this difference in interface thermal properties comes because of the difference in thermal conductivity of the buffer layers. Recent studies on AlGaN/GaN high-electron-mobility transistors grown on different substrates indicated that the thermal conductivities of both the substrate and the buffer layer (AlN, for example) has a crucial role in attaining a low TBR [50] , [51] . In these structures, the poor crystal quality of the AlN and associated low thermal conductivity were shown to restrict heat transfer from the GaN into the substrate, leading to high TBR values. A numerical study on the self-heating effects of oxide-confined vertical-cavity surface emitting lasers gives further evidence that the oxide layer, due to its low thermal conductivity, strongly suppresses the heat flow [52] . Therefore, higher T j and R th associated with the device grown with SiO 2 buffer layer could be attributed to additional TBR added to the GaN/sapphire interface negating the benefits offered by the improved crystal quality. It should be remembered that the GaN/sapphire interface itself is characterized by a high degree of TBR in the order of 10 −7 m 2 K W −1 owing to the poor thermal and lattice mismatch between the two layers [53] . Even higher TBR can be expected in practical devices depending on the quality of the nucleation layer (presently low-temperature grown AlN or GaN is used as a nucleation layer) and the extent of interface disorder. It is, therefore, essential that the heat be sufficiently spread out in the GaN layer before crossing the GaN/sapphire boundary; if not, the TBR may entail larger thermal consequences. In order for this to happen, the GaN crystal quality should be sufficiently high with low number of dislocations. Although the lateral overgrowth of GaN on SiO 2 micropatterns can result in high crystal quality, the poor thermal conductivity of the SiO 2 restricts the heat flow across the interface, as evidenced from the results. In light of the above, it is quite plain that the relatively high thermal conductivity of rGO and its associated rapid heat-spreading ability [23] , [29] has a key role in reducing the T j and R th for the devices grown on rGO pattern. It is noteworthy to mention here that the graphene with many materials offers a low TBR in the order of 10 −8 m 2 K W −1 ( [40] ), which is more than an order of magnitude lower than the reported TBR at the GaN/sapphire interfaces. With rGO embedded at the interface between the GaN and sapphire, one can, therefore, assume an effective TBR of about an order of magnitude less compared with the one usually present at the GaN/sapphire interface. The mechanism can be understood by considering the far better GaN/rGO interface than the GaN/sapphire interface in terms of GaN structural quality and thermal conductivity of the buffer layer (see Supplementary Fig. S6 ). In other words, the heat spreading within the GaN as a result of enhanced crystal quality and by the embedded rGO pattern, as well as the improved heat transfer to the sapphire through the rGO due to low TBR, should account for the observed heat dissipation in the GaN LEDs. In summary, we have demonstrated the experimental realization of GaN-based LEDs with embedded graphene oxide pattern for effective heat removal. Scalable graphene oxide microscale pattern has been generated by using a combination of facile lithography and spray-coating methods. The appealing versatility is that the generated graphene oxide pattern acts as a buffer layer for the epitaxial lateral overgrowth of single-crystal high-quality GaN in the fabrication of graphene oxide-embedded devices, which offered excellent heat dissipation while maintaining electrical and optical properties superior to that of its conventional counterpart. Experiments performed in parallel with an SiO 2 buffer layer reveal that the heat dissipation perceived in graphene oxide-embedded device stems not only from graphene’s envisaged lateral heat spreading but also likely from its assenting impact on the TBR at the GaN/sapphire interface. This study comprising of facile approaches to unravel the heat dissipation issues in LED imparts the potential of graphene in optoelectronic devices for a better thermal management. Our findings may, therefore, instigate yet new discoveries that eventually make roads to the development of durable high-power LEDs for the next generation of solid-state lighting. Formation of large-scale graphene oxide pattern We used a commercial graphene oxide dispersion (supplied by graphene supermarket) of concentration 5 g l −1 in our experiments. The graphene oxide film with circular hole arrays was obtained as follows. First, an array of circular photoresist patterns having size and period of 4 and 2 μm, respectively, was made on the 2-inch sapphire using standard photolithography. The graphene oxide dispersion was sprayed onto the substrate using an airbrush system with nitrogen as a carrier gas. The airbrush inlet pressure of nitrogen, substrate temperature and spraying rate were 2 bars, 130 °C and 3 ml min −1 , respectively. The deposition of SiO 2 was carried out in a plasma-enhanced chemical vapour-deposition system on a similarly photoresist-patterned sapphire substrate. The photoresist was subsequently removed by using acetone, and the resultant graphene oxide and SiO 2 buffer-layer-covered substrates were cleaned with methanol and deionized water, before being set into an AIXTRON RF200 horizontal metal-organic chemical vapour deposition reactor. Fabrication of rGO- and SiO 2 -embedded GaN LEDs In the metal-organic chemical vapour deposition reactor, first step was the thermal annealing process at 1100 °C with hydrogen carrier gas for the reduction of graphene oxide and thermal cleaning of sapphire substrate. The next step was the deposition of a GaN nucleation layer at 560 °C under a pressure of 400 mbar. Trimethylgallium and ammonia were used as the gallium and nitrogen sources, respectively. Then the growth of undoped GaN layer was conducted at a high temperature in two successive steps. In the first step, the temperature and pressure were maintained at 1050 °C and 500 mbar, respectively, whereas in the second step the values of the respective parameters were increased to 1120 °C and 100 mbar to get high lateral growth and planarize the epilayer. Following this step, a 2-μm silicon-doped n-type GaN template, five-period multiquantum wells of InGaN/GaN pairs at 860 °C and a 110 nm magnesium-doped p-GaN layer at 1050 °C were grown in succession to complete the fabrication of rGO- or SiO 2 -embedded LED structure. Mesa etching was carried out using standard photolithography and inductively coupled plasma reactive ion etching. Finally, Cr/Ni/Au and Ni/Au metal stacks were deposited by e-beam evaporation to serve as respective metal pads to the n- and p-type layers. Characterization The surface topography of the graphene oxide pattern was probed by AFM (Digital Instruments; Nanoscope IV A) in tapping mode. X-ray photoelectron spectroscopy (AXIS-Nova, Kratos) measurements were recorded in an ultrahigh vacuum chamber (7 × 10 −9 torr) using Al K α radiation (1486.6 eV). X-ray diffraction (X’PERT-MRD) and scanning electron microscopy (HITACHI-S-4300SE) analyses were performed to understand the growth behaviour and the quality of GaN directly grown on the rGO pattern. TEM (FEI, Techani G 2 300 KeV) was used to verify the existence of rGO at the interface of sapphire/GaN and to study the crystal quality of GaN. The surface temperature distribution and peak temperature of the LED chips were examined using infrared thermal imaging camera (FLIR Thermovision A40M thermal imager). The thermal sensitivity of the camera was better than 0.08 °C and had a spatial resolution of 50 μm while operating in the spectral range from 7.5–13 μm. The thermal transient measurements were carried out in a thermal transient tester (T3ster, MicRed). For this measurement, LED packages (SMD type, product no. 2076-4, supplied by Tato, Taiwan) consisting of chips of dimension 600 × 600 μm 2 were used. Silver paste was used for mounting the chips on an aluminium heat-sink. The theoretical framework of the evaluation of the T3ster is based on a representation of the distributed RC networks. After a calibration process, which determines the ratio between the forward voltage drop as a temperature-sensitive parameter and temperature, transient cooling curve was measured for different injection currents. The structure functions were obtained by direct mathematical transformations from the transient cooling curves. Current-voltage and light-output-current measurements were carried out using a probe station system. How to cite this article: Han, N. et al. Improved heat dissipation in gallium nitride light-emitting diodes with embedded graphene oxide pattern. Nat. Commun. 4:1452 doi: 10.1038/ncomms2448 (2013).